ASK3 responds to osmotic stress and regulates blood pressure by suppressing WNK1-SPAK/OSR1 signaling in the kidney Changes in the osmolality of body fluids pose a serious danger to cells and living organisms, which have developed cellular systems to sense and respond to osmotic stress and to maintain homoeostasis of body fluid. However, these processes are incompletely understood in mammals. Here we show that apoptosis signal-regulating kinase 3 (ASK3) is predominantly expressed in the kidney and alters its kinase activity bidirectionally in response to osmotic stress. We further demonstrate that ASK3 interacts with WNK1, mutation in which causes an inherited form of hypertension in humans. Knockdown of Ask3 by short interfering RNA enhances the activation of the WNK1-SPAK/OSR1 signalling pathway. Moreover, Ask3 knockout mice exhibit a hypertensive phenotype, in addition to hyperactivation of SPAK/OSR1 in renal tubules. Our results suggest that ASK3 is a unique bidirectional responder to osmotic stress and that it has a role in the control of blood pressure as an upstream suppressor of the WNK1-SPAK/OSR1 signalling pathway. The maintenance of the fluid balance is one of the most important issues for organisms. Thus, all living organisms are equipped with systems that sense and respond to osmolality at the cellular level [1] , [2] . Both hypotonic and hypertonic situations are serious stress for cells, resulting in the perturbation of various cell functions, such as cell adhesion, gene expression, proliferation and apoptosis [1] , [2] , [3] , [4] . Cells must transduce not only the ‘quantity’ but also the ‘direction’ of the osmotic changes to maintain osmotic homoeostasis. Several signal transduction pathways have been proposed to be involved in either the hypertonic or hypotonic stress response [1] , [2] , [4] . However, because there have been few studies that deal with osmolality as a graded amount of stress throughout a range from hypotonic to hypertonic situations, it is largely unknown whether and, if so, how a common machinery can manage both osmotic stresses. The mitogen-activated protein kinase (MAPK) cascades are one of the major pathways regulating osmotic stress response and are well conserved from yeast to humans [1] , [5] , [6] . Activated MAPK induces various stress responses, such as gene expression and apoptosis [7] , [8] . Several MAP kinase kinase kinases (MAP3Ks), including MEKK2, MEKK3 and TAK1, have been reported to become activated in hypertonic stress to initiate the MAPK cascade in mammalian cells [9] , [10] . However, little is known about the activation mechanisms and physiological roles of these MAP3Ks in osmotic stress responses. Furthermore, the involvement of other MAP3Ks in osmotic stress response is still elusive in mammals. Recently, with-no-lysine [K] 1 (WNK1), which belongs to a unique kinase family, has been proposed to regulate the osmotic stress response [11] , [12] . Activated by osmotic stress, WNK1 phosphorylates and activates STE20/SPS1-related proline/alanine-rich kinase (SPAK) and oxidative stress-responsive kinase 1 (OSR1) [13] , [14] . These two downstream kinases regulate ion transporters that control the cell volume [15] , [16] , [17] . The WNK1-SPAK/OSR1 pathway is also proposed to function in renal salt reabsorption and blood pressure control [12] , [14] , [17] . The WNK1 gene mutation, which causes overexpresssion of the WNK1 protein and misregulation of its splicing, results in an inherited hypertension termed pseudohypoaldosteronism type II (PHA II) in humans [18] , [19] , [20] , presumably due to excess NaCl reabsorption in the renal tubules [12] , [20] . Thus, the WNK1-SPAK/OSR1 pathway, which is activated by osmotic stress, appears to be involved in the pathogenesis of inherited hypertension and might be a cue to integrate the cellular osmotic response into the control of systemic blood pressure. However, it is still unclear how the activity of the WNK1-SPAK/OSR1 pathway is regulated by osmotic stress and whether the hypertensive phenotype induced by WNK1 mutation is attributable to the misregulation of the WNK1-SPAK/OSR1 pathway. In the present study, we demonstrate that a newly characterized MAP3K, apoptosis signal-regulating kinase 3 (ASK3) [21] , is activated and inactivated by hypotonic and hypertonic stress, respectively. We also found that ASK3 interacted with WNK1 and inhibited the WNK1-SPAK/OSR1 pathway in a kinase activity-dependent manner. Consistent with these results, ASK3 knockout mice exhibited hyperactivation of SPAK/OSR1 and Na + –Cl − cotransporter (NCC) in the renal tubules, in addition to suffering from mild hypertension. Our results suggest that ASK3 is a unique bidirectional responder to both hypo- and hyper-tonic stress and that it functions as an upstream suppressor of the WNK1-SPAK/OSR1 pathway in the kidney to control the systemic blood pressure. ASK3 is predominantly expressed in the kidney To find new kinases involved in stress response, we performed a database search based on homology with ASK1 (MAP3K5) [22] . We determined that MAP3K15 is highly homologous to ASK1 and ASK2 (MAP3K6), and thus, we have named MAP3K15 as ‘ASK3’ ( Fig. 1a ) [21] . Because ASK1 and ASK2 have been reported to activate the JNK and p38 MAPK pathways [22] , [23] , we examined whether ASK3 also functions as a MAP3K. Similar to ASK1, overexpression of ASK3 WT but not a kinase-negative mutant of ASK3 (ASK3 KM) activated both JNK and p38 but not ERK ( Fig. 1b ), suggesting that ASK3 serves as a MAP3K of the JNK and p38 pathways. 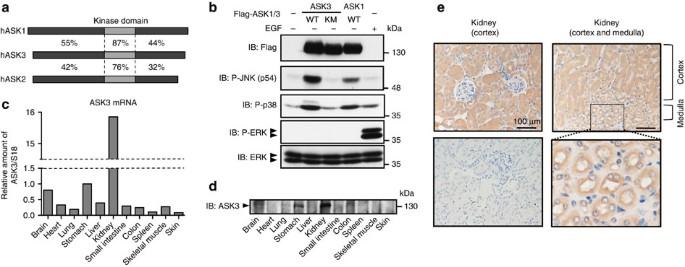Figure 1: The properties of ASK3 as an ASK family protein with a unique tissue distribution. (a) Schematic drawings of the ASK family kinases. The identity of the amino-acid sequences of human ASK3 (hASK3) with hASK1 and hASK2 are indicated in the N-terminus, the kinase domain and the C-terminus. (b) The activation of MAPKs due to the overexpression of ASK constructs was analysed by immunoblotting (IB). Epidermal growth factor (EGF) was applied as a positive control for ERK activation. (c) A real-time quantitative PCR for ASK3 mRNA in various tissues. The amount was normalized to the mRNA of S18 ribosomal protein as an internal control, and the relative amount to that in stomach are shown. (d) A tissue immunoblot analysis of ASK3. Tissue lysates containing equal amount of total protein (150 μg protein per lane) were immunoprecipitated with ASK3 antibody, and then detected by IB. (e) Immunohistochemical staining of ASK3 in the kidney. The ASK3 signals were visualized by DAB staining (brown). The lower left panel shows a negative control treated with control IgG. The lower right panel represents a magnified image of the square in the upper panel. Scale bar, 100 μm. Figure 1: The properties of ASK3 as an ASK family protein with a unique tissue distribution. ( a ) Schematic drawings of the ASK family kinases. The identity of the amino-acid sequences of human ASK3 (hASK3) with hASK1 and hASK2 are indicated in the N-terminus, the kinase domain and the C-terminus. ( b ) The activation of MAPKs due to the overexpression of ASK constructs was analysed by immunoblotting (IB). Epidermal growth factor (EGF) was applied as a positive control for ERK activation. ( c ) A real-time quantitative PCR for ASK3 mRNA in various tissues. The amount was normalized to the mRNA of S18 ribosomal protein as an internal control, and the relative amount to that in stomach are shown. ( d ) A tissue immunoblot analysis of ASK3. Tissue lysates containing equal amount of total protein (150 μg protein per lane) were immunoprecipitated with ASK3 antibody, and then detected by IB. ( e ) Immunohistochemical staining of ASK3 in the kidney. The ASK3 signals were visualized by DAB staining (brown). The lower left panel shows a negative control treated with control IgG. The lower right panel represents a magnified image of the square in the upper panel. Scale bar, 100 μm. Full size image Different from the expression pattern of ASK1 or ASK2 (ref. 24 ), ASK3 was predominantly detected in the kidney by real-time quantitative PCR analysis ( Fig. 1c ) and immunoblot analysis probed with an ASK3-specific antibody ( Fig. 1d and Supplementary Fig. S1a ). In the mouse kidney, ASK3 was expressed in the epithelium of the renal tubules in both the cortex and the medulla but not in the glomeruli ( Fig. 1e ). Interestingly, the ASK3 signal was localized around the apical lumen of renal epithelial cells in the medulla. We also confirmed the presence of the ASK3 transcript in the renal tubules by in situ hybridization ( Supplementary Fig. S2 ). These findings suggested that ASK3 is expressed in renal epithelial cells that are directly exposed to the massive osmotic changes in the kidney. ASK3 responds bidirectionally to osmotic stress According to the tissue distribution, we examined whether ASK3 responds to the osmotic stress. We monitored the kinase activity of endogenous ASK3 in HEK293A cells using a P-ASK antibody [25] (see Supplementary Figs S1c and S3 for detailed information about the P-ASK antibody) after changing the culture medium to hypo- (200 mOsm), iso- (300 mOsm) or hyper- (500 mOsm) osmotic solutions ( Fig. 2a ). Intriguingly, ASK3 exhibited moderate basal activity in isotonic solution and was activated and inactivated in the hypotonic and hypertonic stress, respectively. The osmolality dependency of the kinase activity was further confirmed by the in vitro kinase assay ( Supplementary Figs S3d and S4 ). We also investigated the osmotic response of other ASK isoforms using the P-ASK antibody. ASK2 but not ASK1 showed similar bidirectional response to osmotic stress ( Supplementary Fig. S5 ). To investigate how sensitively ASK3 responds to osmotic changes, we gradually altered the concentration of NaCl by 10-mM steps ( Fig. 2b ) or mannitol by 20-mM steps ( Supplementary Fig. S6 ) in the extracellular solutions. The kinase activity of ASK3 was affected in both directions by a 10–20 mOsm change around the isotonic condition (130 mM NaCl). Both the activation in hypotonic stress and the inactivation in hypertonic stress occurred as early as 2 min after the osmolality changes ( Fig. 2c ). Furthermore, the activity of ASK3 was reversed within 10 min by the inversion of the osmotic stress ( Fig. 2d ). These results suggest that the activity of ASK3 is tightly regulated by osmolality in a sensitive, rapid and reversible manner. 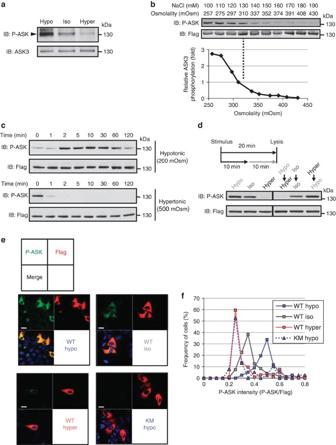Figure 2: ASK3 responds bidirectionally to osmotic stress. (a) The osmotic response of endogenous ASK3. ASK3 was immunoprecipitated from HEK293A cells and its kinase activity was evaluated by immunoblotting (IB) using a P-ASK antibody. (b) The NaCl concentration of the extracellular solutions was gradually altered in 10-mM steps. The actual osmolality of the solutions measured by osmometer are shown under the NaCl concentrations. The relative ASK3 activity was normalized to the value at 130 mM NaCl (isotonic). (c) The time course of ASK3 activity in response to osmotic stress. (d) The reversibility of ASK3 activity. HEK293A cells were exposed to the indicated osmotic solution for 20 min in the three lanes on the left. In the three lanes on the right, the solution was exchanged at the halfway point (10 min). (e) The confocal images of double immunofluorescence with P-ASK (green) and Flag (red) in HEK293A cells transfected with Flag-ASK3 WT or Flag-ASK3 KM. Cells were exposed to the indicated osmotic solutions for 20 min before the fixation. Scale bar, 20 μm. (f) The frequency distribution of the P-ASK/Flag ratio derived from the immunofluorescence images under conditions similar to those of panele. The Flag signal-positive cells were analysed by an image analyser (ArrayScan) to calculate the P-ASK/Flag signal ratio in each cell (n=38–120). Figure 2: ASK3 responds bidirectionally to osmotic stress. ( a ) The osmotic response of endogenous ASK3. ASK3 was immunoprecipitated from HEK293A cells and its kinase activity was evaluated by immunoblotting (IB) using a P-ASK antibody. ( b ) The NaCl concentration of the extracellular solutions was gradually altered in 10-mM steps. The actual osmolality of the solutions measured by osmometer are shown under the NaCl concentrations. The relative ASK3 activity was normalized to the value at 130 mM NaCl (isotonic). ( c ) The time course of ASK3 activity in response to osmotic stress. ( d ) The reversibility of ASK3 activity. HEK293A cells were exposed to the indicated osmotic solution for 20 min in the three lanes on the left. In the three lanes on the right, the solution was exchanged at the halfway point (10 min). ( e ) The confocal images of double immunofluorescence with P-ASK (green) and Flag (red) in HEK293A cells transfected with Flag-ASK3 WT or Flag-ASK3 KM. Cells were exposed to the indicated osmotic solutions for 20 min before the fixation. Scale bar, 20 μm. ( f ) The frequency distribution of the P-ASK/Flag ratio derived from the immunofluorescence images under conditions similar to those of panel e . The Flag signal-positive cells were analysed by an image analyser (ArrayScan) to calculate the P-ASK/Flag signal ratio in each cell ( n =38–120). Full size image We suspected that the progressive change of the P-ASK signal in the immunoblot analysis might be merely due to the change in the number of cells that exhibit a certain activity of ASK3 in the population. To examine whether a gradual change in the phosphorylation of ASK3 occurs at a single-cell level, we performed an immunocytochemical analysis using a newly generated P-ASK antibody (PA41) ( Supplementary Fig. S1c ). The P-ASK signal was gradually altered depending on the osmotic stress in each cell transfected with Flag-ASK3 WT ( Fig. 2e ). We could not detect any P-ASK signal in the cells transfected with Flag-ASK3 KM even under a hypotonic stress condition, suggesting that the phosphorylation of ASK3 relies on its own kinase activity. Furthermore, to assess the degree of ASK3 activity more quantitatively, we calculated the ratio of phospho-signal to total protein signal (P-ASK/Flag) in each cell using an image analyser (ArrayScan; Thermo Scientific Cellomics). A comparison of the frequency distribution of the ratio under the different osmotic conditions showed that the phosphorylation of ASK3 was gradually changed in each cell ( Fig. 2f ), confirming that ASK3 is a bidirectional responder to osmotic stress. ASK3 regulates the WNK1-SPAK/OSR1 signalling pathway To explore the role of ASK3 in the kidney, we performed a yeast two-hybrid screen of a human kidney cDNA library and identified WNK1 as an ASK3-binding protein. WNK1 is a Ser/Thr kinase with a unique kinase domain [11] that has recently been reported to regulate diverse ion cotransporters and channels that are involved in the control of cell volume and blood pressure. Moreover, it has also been reported that the kinase activity of WNK1 is altered by osmotic stress [12] , [14] , [26] . Therefore, we investigated the relationship between ASK3 and WNK1 in human cells. Endogenous WNK1 was coimmunoprecipitated with ASK3 in HEK293F cells, confirming the interaction between ASK3 and WNK1 ( Fig. 3a ). The interaction was not affected by the osmotic conditions ( Fig. 3b ). The kinase activity of coimmunoprecipitated ASK3 showed a bidirectional response as is described in Fig. 2a , suggesting that ASK3 and WNK1 form a stable complex independently from the ASK3 activity. Other ASK isoforms were also coimmunoprecipitated with WNK1 ( Supplementary Fig. S7 ). 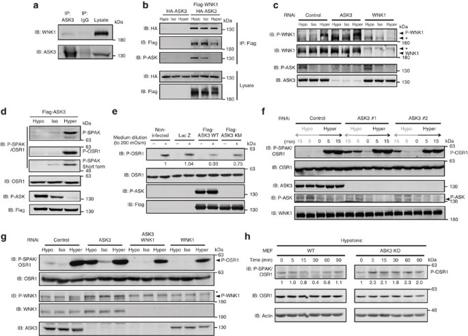Figure 3: ASK3 suppresses the WNK1-SPAK/OSR1 pathway through its kinase activity. (a) Coimmunoprecipitation of endogenous WNK1 with ASK3 in HEK293F cells. (b) Coimmunoprecipitation of HA-ASK3 with Flag-WNK1 under the hypo-, iso- and hyper-tonic conditions. (c) The indicated siRNAs were transfected into HEK293A cells, and cells were exposed to each osmotic stress for 10 min. The cell lysates were analysed by immunoblotting (IB) using phospho-specific antibodies to monitor the kinase activities of WNK1 and ASK3. The asterisks (*) indicate nonspecific bands. (d) HEK293A cells were transfected with Flag-ASK3 and exposed to solutions of varying osmolarity. The activities of endogenously expressed SPAK and OSR1 were analysed by IB using a P-SPAK/OSR1 antibody. (e) HeLa cells were infected with adenovirus (100 MOI) encoding Lac Z, Flag-ASK3 WT or Flag-ASK3 KM to overexpress these proteins. The cells were exposed to diluted medium (200 mOsm) for 10 min. The quantified relative amounts of P-OSR1 are indicated below the bands. (f) HeLa cells were transfected with a control or two independent ASK3 siRNAs, followed by the treatment with both hypo- and hypertonic solutions for the indicated durations. (g) HeLa cells were transfected with a single siRNA or a combination of siRNAs (ASK3+WNK1). The cells were treated with both hypo- and hyper-tonic solutions for 15 min. * indicates nonspecific bands. (h) MEFs derived from WT or ASK3 KO mice were exposed to hypotonic stress for the indicated durations. The intensity of P-OSR1 signal was quantified by densitometry and shown under the bands (normalized to each intensity at time 0). Figure 3: ASK3 suppresses the WNK1-SPAK/OSR1 pathway through its kinase activity. ( a ) Coimmunoprecipitation of endogenous WNK1 with ASK3 in HEK293F cells. ( b ) Coimmunoprecipitation of HA-ASK3 with Flag-WNK1 under the hypo-, iso- and hyper-tonic conditions. ( c ) The indicated siRNAs were transfected into HEK293A cells, and cells were exposed to each osmotic stress for 10 min. The cell lysates were analysed by immunoblotting (IB) using phospho-specific antibodies to monitor the kinase activities of WNK1 and ASK3. The asterisks (*) indicate nonspecific bands. ( d ) HEK293A cells were transfected with Flag-ASK3 and exposed to solutions of varying osmolarity. The activities of endogenously expressed SPAK and OSR1 were analysed by IB using a P-SPAK/OSR1 antibody. ( e ) HeLa cells were infected with adenovirus (100 MOI) encoding Lac Z, Flag-ASK3 WT or Flag-ASK3 KM to overexpress these proteins. The cells were exposed to diluted medium (200 mOsm) for 10 min. The quantified relative amounts of P-OSR1 are indicated below the bands. ( f ) HeLa cells were transfected with a control or two independent ASK3 siRNAs, followed by the treatment with both hypo- and hypertonic solutions for the indicated durations. ( g ) HeLa cells were transfected with a single siRNA or a combination of siRNAs (ASK3+WNK1). The cells were treated with both hypo- and hyper-tonic solutions for 15 min. * indicates nonspecific bands. ( h ) MEFs derived from WT or ASK3 KO mice were exposed to hypotonic stress for the indicated durations. The intensity of P-OSR1 signal was quantified by densitometry and shown under the bands (normalized to each intensity at time 0). Full size image We next examined the mutual regulation of kinase activities between ASK3 and WNK1. The kinase activity of WNK1 was monitored by immunoblotting with a phospho-specific antibody (P-Ser 382 in WNK1) as reported previously [27] . Consistent with previous reports [12] , [27] , [28] , WNK1 was activated by hypertonic stress in control siRNA-treated cells ( Fig. 3c and Supplementary Fig. S8 ), indicating that the kinase activity of WNK1 is oppositely regulated to that of ASK3 in response to hypertonic stress. When endogenous ASK3 was depleted by siRNA, the kinase activity of WNK1 was enhanced. In contrast, WNK1 depletion did not yield any detectable effect on the ASK3 activity ( Fig. 3c ). These results suggest that ASK3 functions as an upstream regulator of WNK1 to suppress its kinase activity. WNK1 phosphorylates and activates SPAK and OSR1 [14] . These two downstream kinases are known to regulate ion transporters in the osmotic stress response [15] , [16] , [17] . We generated a phospho-specific antibody to a conserved WNK1-mediated phosphorylation site of SPAK and OSR1 (P-SPAK/OSR1) ( Supplementary Fig. S1d,e ) (Thr 233 and Thr 185 in SPAK and OSR1, respectively) [14] , [27] and examined the response of SPAK/OSR1 to osmotic stress. In HEK293A cells, SPAK and OSR1 were activated by hypertonic stress, and SPAK was inactivated by hypotonic stress, which was the reciprocal pattern of the activity of ASK3 ( Fig. 3d ), implying that ASK3 may function as a negative regulator of the WNK1-SPAK/OSR1 pathway in a kinase activity-dependent manner. We further examined the relationship between ASK3 and the WNK1-SPAK/OSR1 pathway in HeLa cells, in which a tight regulation of OSR1 activity by WNK1 had been reported [15] , [27] . We found that the overexpression of ASK3 WT, but not of ASK3 KM, strongly suppressed the activity of OSR1 in hypotonic stress ( Fig. 3e ), suggesting that ASK3 inhibits OSR1 in a kinase activity-dependent manner. ASK3 depletion by two independent siRNAs resulted in the acceleration of OSR1 activity, particularly in hypotonic stress rather than in hypertonic stress ( Fig. 3f ), which is consistent with the hypothesis that ASK3 suppresses OSR1 with its kinase activity. The P-ASK signal was reduced but still observed under the ASK3 depletion, which appeared to be derived from other ASK isoforms ( Supplementary Fig. S9a ). However, either depletion of ASK1 or ASK2 had marginal effect on OSR1 activity ( Supplementary Fig. S9b ). Moreover, an additional depletion of ASK1 and ASK2 together with ASK3 (ASK triple knock down) did not lead to further activation of OSR1 than ASK3 single depletion ( Supplementary Fig. S9a ). These results suggested that ASK3 may have a pivotal role in the regulation of OSR1 activity among ASK isoforms. The downstream MAPKs, JNK and p38 ( Fig. 1b ), did not seem to be involved in the regulation of the WNK1-SPAK/OSR1 pathway, because the inhibitors of JNK and p38 did not enhance the OSR1 activity in response to hypotonic stress as ASK3 depletion did ( Supplementary Fig. S10 ). To examine whether ASK3 inhibits OSR1 activity through the suppression of WNK1, we performed a combinatorial knockdown of ASK3 and WNK1 ( Fig. 3g ). In the control knockdown cells, OSR1 was activated slightly and strongly by hypotonic and hypertonic stress, respectively. The activation of OSR1 was suppressed by the depletion of WNK1 alone, confirming the previous report that WNK1 is a major activator of OSR1 in osmotic stress [27] . In ASK3-depleted cells, OSR1 was strongly activated not only by hypertonic stress but also by hypotonic stress, which was consistent with the WNK1 activity monitored by P-WNK1 signal ( Fig. 3g ). The hypotonic stress-induced activation of OSR1 was completely abolished by the additional depletion of WNK1 with ASK3 knockdown. These results suggest that the hypotonicity-induced OSR1 hyperactivation in the absence of ASK3 was mediated by the misregulation of WNK1. The hyperactivation of endogenous WNK1 under ASK3 depletion was confirmed by an in vitro kinase assay ( Supplementary Fig. S11 ). On the other hand, we found that other WNK family kinases (WNK2-4), among which WNK3 and WNK4 have been reported to activate SPAK/OSR1 (ref. 29 ), were also coimmunoprecipitated with ASK3 ( Supplementary Fig. S12a ). However, the depletion of WNK1 showed more dominant effect than those of other WNK isoforms on the OSR1 activity ( Supplementary Fig. S12b ). The result endorses the notion that the hyperactivation of OSR1 upon ASK3 depletion is mainly regulated through the WNK1 misregulation. We further examined the hypotonic stress response of OSR1 in mouse embryonic fibroblasts (MEFs) derived from WT and ASK3 KO mice ( Supplementary Fig. S13 ). Consistent with the result of ASK3-knockdown HeLa cells, the activation of OSR1 was accelerated in ASK3 KO MEFs ( Fig. 3h ). The hyperactivation of OSR1 in ASK3 KO MEFs was suppressed by the exogenous ASK3 expressed via the adenovirus infection ( Supplementary Fig. S14 ). These results further supported the hypothesis that ASK3 functions as a suppressor of the WNK1-OSR1 pathway in hypotonic stress. ASK3 knockout mice exhibit a hypertensive phenotype A mutation of WNK1 gene, which leads to the overexpression of the WNK1 protein and the misregulation of its splicing, has been reported to be a cause of a hereditary hypertension termed PHA II [18] , [30] . This pathogenic mutation has been considered to eventually cause hypertension through the hyperactivation of NCC and Na + -K + -2Cl - cotransporter (NKCC), the substrates of SPAK/OSR1 (refs 12 , 16 , 18 , 19 , 20 , 31 ). Furthermore, it has recently been demonstrated in vivo that the SPAK activity that is regulated by WNK kinases is physiologically important for controlling the blood pressure through the regulation of the renal ion transporters NCC and NKCC [32] . Considering the suppressive function of ASK3 on the WNK1-SPAK/OSR1 pathway together with the fact that ASK3 is also expressed in the kidney ( Fig. 1c–e ), we speculated that ASK3 might regulate the WNK1-SPAK/OSR1-NCC pathway in renal tubules to control the systemic blood pressure. Thus, we next examined the activity of SPAK/OSR1 and of its substrate NCC in the renal tubules of ASK3 KO mice. The immunostaining of serial cryosections of the renal cortex with P-SPAK/OSR1, total NCC (T-NCC) and phospho-NCC (P-NCC) [33] antibodies suggested that the serial renal tubules labelled by the T-NCC antibody (the distal convoluted tubules, or DCT) were properly detected by the P-SPAK/OSR1 and P-NCC antibodies ( Fig. 4a ). Additionally, the P-SPAK/OSR1 and P-NCC but not T-NCC signals disappeared after treatment with λ-phosphatase ( Supplementary Fig. S15 ), confirming the phospho-specificity of these antibodies. In the renal cortex of ASK3 KO mice, the P-SPAK/OSR1 signals were stronger and the number of signal-positive tubules was increased compared with those of WT mice ( Fig. 4b ). We objectively quantified the confocal images using the image analyser ArrayScan ( Supplementary Fig. S16 ). The area of the signal-positive region was significantly increased in the ASK3 KO mice ( Fig. 4c ). These results suggest that the genetic depletion of ASK3 enhanced the SPAK/OSR1 activity and increased the area of SPAK/OSR1-active renal tubules in the kidney. We performed a similar analysis of the immunofluorescence images probed with T-NCC and P-NCC. In the ASK3 KO mice, the expression area of NCC (labelled with the T-NCC antibody) was not altered ( Fig. 4d ), and the P-NCC-positive area was slightly, but not significantly, increased ( Fig. 4e ). To totally evaluate the NCC activity at the whole-kidney level, we performed an immunoblot analysis in the kidney lysate with the P-NCC antibody. The P-NCC intensity was modestly but significantly increased in the kidneys of ASK3 KO mice compared with those of WT mice without any alteration in the protein levels of WNK1 or OSR1 ( Fig. 4f ). These results suggest that ASK3 functions as a suppressor of SPAK/OSR1 and thus NCC in the DCT of the mouse kidney. 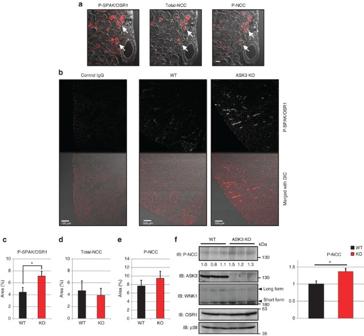Figure 4: SPAK/OSR1 and NCC is hyperactivated in the kidney of ASK3 knockout mice. (a) Immunofluorescence images of serial cryosections of the mouse kidney probed with P-SPAK/OSR1, total-NCC and P-NCC antibodies. The representative signals (shown in red) in serial renal tubules are indicated by white arrows. The differential interference contrast (DIC) images are merged. Scale bar, 20 μm. (b) Low-power immunofluorescence images of the kidney probed by control IgG (left) and P-SPAK/OSR1 (middle: WT, right: ASK3 KO). The lower panels show the images merged with the DIC (the fluorescence signals are shown in red). Scale bar, 100 μm. (c–e) The fractions of the areas that are immunostained by each antibody were quantified by an image analyser (black bar, WT:n=3; red bar, ASK3 KO:n=3,P=0.026 inFig. 3c); Data are means±s.e.m. (details are described inSupplementary Fig. S16). *Pis for a two-sidedt-test comparing WT with ASK3 KO. (f) The kidney lysate of WT and ASK3 KO mice were analysed by immunoblotting with the described antibodies. The quantified relative amounts of P-NCC are indicated below the bands and summarized in a bar graph (black bar, WT:n=3; red bar, ASK3 KO:n=3,P=0.048); The data are represented as the means±s.e.m. *Pis for a two-sidedt-test comparing WT with ASK3 KO. Figure 4: SPAK/OSR1 and NCC is hyperactivated in the kidney of ASK3 knockout mice. ( a ) Immunofluorescence images of serial cryosections of the mouse kidney probed with P-SPAK/OSR1, total-NCC and P-NCC antibodies. The representative signals (shown in red) in serial renal tubules are indicated by white arrows. The differential interference contrast (DIC) images are merged. Scale bar, 20 μm. ( b ) Low-power immunofluorescence images of the kidney probed by control IgG (left) and P-SPAK/OSR1 (middle: WT, right: ASK3 KO). The lower panels show the images merged with the DIC (the fluorescence signals are shown in red). Scale bar, 100 μm. ( c – e ) The fractions of the areas that are immunostained by each antibody were quantified by an image analyser (black bar, WT: n =3; red bar, ASK3 KO: n =3, P =0.026 in Fig. 3c ); Data are means±s.e.m. (details are described in Supplementary Fig. S16 ). * P is for a two-sided t -test comparing WT with ASK3 KO. ( f ) The kidney lysate of WT and ASK3 KO mice were analysed by immunoblotting with the described antibodies. The quantified relative amounts of P-NCC are indicated below the bands and summarized in a bar graph (black bar, WT: n =3; red bar, ASK3 KO: n =3, P =0.048); The data are represented as the means±s.e.m. * P is for a two-sided t -test comparing WT with ASK3 KO. Full size image It has been demonstrated that the hyperactivation of the SPAK/OSR1-NCC pathway leads to systemic hypertension through the excess reabsorption of NaCl in the DCT [17] , [32] , [34] . Therefore, we measured the blood pressure of ASK3 KO mice by a tail-cuff method. The systolic blood pressure (SBP) of the ASK3 KO littermates (SBP: 105.9±1.8 mm Hg) was similar to that of WT (105.9±2.1 mm Hg) at 14 weeks of age. However, the SBP of the ASK3 KO mice increased significantly along with aging, reaching 115.9±3.6 mm Hg at 30 weeks, whereas that of the WT mice was only slightly increased (109.3±1.5 mm Hg) at the same age ( Fig. 5a ). 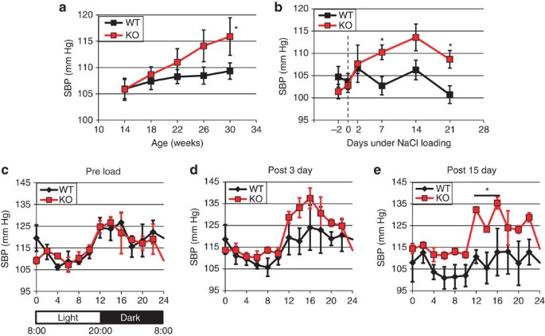Figure 5: ASK3 knockout mice exhibit a hypertensive phenotype. (a) The SBP of WT and ASK3 KO littermates (black square, WT:n=14; red square, ASK3 KO:n=9–10,P=0.018) at the indicated ages. The data are represented as the means±s.e.m. *P-value is for a two-sidedt-test comparing the SBP at 30 weeks with that at 14 weeks. (b) The changes in the SBP after dietary NaCl loading. The SBP was measured on the indicated days of NaCl loading (black square, WT:n=6; red square, ASK3 KO:n=7-8,P=0.010 for 7th day andP=0.010 for 21st day); The data are represented as the means±s.e.m. *P-value is for a two-sidedt-test comparing the SBP of the ASK3 KO with that of the WT at the same day. (c–e) The telemetry measurement of the SBP before loading (Pre load) and 3 and 15 days after the start of NaCl loading (black square, WT:n=3; red square, ASK3 KO:n=3). Data are obtained every minute and averaged every 2 h. The light and dark periods are indicated by the white and black bars, respectively. *P=0.045 for a two-sidedt-test comparing the SBP of the ASK3 KO with that of the WT at the first half of the dark period of 15th day; The data are represented as the means±s.e.m. Figure 5: ASK3 knockout mice exhibit a hypertensive phenotype. ( a ) The SBP of WT and ASK3 KO littermates (black square, WT: n =14; red square, ASK3 KO: n =9–10, P =0.018) at the indicated ages. The data are represented as the means±s.e.m. * P -value is for a two-sided t -test comparing the SBP at 30 weeks with that at 14 weeks. ( b ) The changes in the SBP after dietary NaCl loading. The SBP was measured on the indicated days of NaCl loading (black square, WT: n =6; red square, ASK3 KO: n =7-8, P =0.010 for 7th day and P =0.010 for 21st day); The data are represented as the means±s.e.m. * P -value is for a two-sided t -test comparing the SBP of the ASK3 KO with that of the WT at the same day. ( c – e ) The telemetry measurement of the SBP before loading (Pre load) and 3 and 15 days after the start of NaCl loading (black square, WT: n =3; red square, ASK3 KO: n =3). Data are obtained every minute and averaged every 2 h. The light and dark periods are indicated by the white and black bars, respectively. * P =0.045 for a two-sided t -test comparing the SBP of the ASK3 KO with that of the WT at the first half of the dark period of 15th day; The data are represented as the means±s.e.m. Full size image We next performed the NaCl loading on the ASK3 KO mice, as excess salt intake is well known to be involved in the pathogenesis of hypertension [35] , [36] . The application of a high-NaCl diet for 21 days significantly increased the SBP of the ASK3 KO mice at the age of 13 weeks (earlier than the spontaneous hypertension, see Fig. 5a ), whereas the SBP of the WT mice was slightly decreased by the same treatment ( Fig. 5b ). This phenotype was unique to ASK3 among ASK isoforms, because neither ASK1 KO nor ASK2 KO mice exhibited hypertension upon the NaCl loading ( Supplementary Fig. S17 ). We further performed telemetry measurement of the blood pressure to more accurately evaluate the salt susceptibility of ASK3 KO mice ( Fig. 5c–e ). Consistent with the result by the tail-cuff method, the SBP of the ASK3 KO mice became significantly higher than that of the WT after NaCl loading in the dark period of 15th day ( Fig. 5e ). The diastolic blood pressure after the NaCl loading was modestly, but not significantly ( P =0.10), higher in the ASK3 KO mice ( Supplementary Fig. S18 ). Together with the result that the ASK3 KO mice showed hyperactivation of SPAK/OSR1 and NCC in the kidney, the hypertensive phenotype of the ASK3 KO mice suggests that ASK3 is involved in blood pressure control, at least in part, through the suppression of the WNK1-SPAK/OSR1 pathway in the renal tubules. Recent studies have revealed that the WNK1-SPAK/OSR1 pathway activates NCC [16] and NKCC [15] and that WNK1 inhibits K + -Cl − cotransporter independent of both SPAK and OSR1 (ref. 26 ) ( Fig. 6 ). Because these transporters have important roles in cell volume regulation and renal salt reabsorption [2] , [17] , WNK1 has received substantial attention in the regulation of the osmotic stress response and systemic blood pressure [12] , [14] . However, little is known about upstream regulators of WNK1 activity. In the present study, we have demonstrated that ASK3 bidirectionally responds to osmotic stress and suppresses the WNK1-SPAK/OSR1 pathway in a kinase activity-dependent manner. The bidirectional alteration of ASK3 activity in a single cell ( Fig. 2e ) may provide a plausible regulation of cellular osmotic response, as cells must respond inversely to oppositely directed stresses (for example, the uptake and excretion of ions) ( Fig. 6 ). Moreover, ASK3 showed a quick response and a reversible flexibility to osmotic stress ( Fig. 2c ), which also appear helpful for the immediate and tight cellular osmotic response. With these properties, we consider that ASK3 may integrate hyper- and hypo-tonic stress responses into a single signal system. 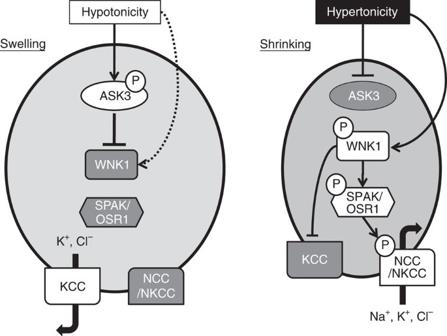Figure 6: A schematic model of ASK3’s role in the cellular osmotic stress response. When a cell is exposed to hypotonic or hypertonic stress, the cell volume is increased (swelling) or decreased (shrinking), respectively. It is broadly understood that various types of ion channels and transporters are regulated by phosphorylation during the restitution of cell volume. K+-Cl−cotransporter (KCC) is activated by the dephosphorylation in response to cell swelling and releases ions to the outside from the cell to decrease the cell volume. In contrast, NKCC is activated by phosphorylation in response to hypertonic stress and imports ions into the cell to increase the cell volume. Our results suggest that hypotonic stress activates ASK3, leading to the inhibition of the WNK1-SPAK/OSR1 pathway. In contrast, hypertonic stress inhibits ASK3, which relieves WNK1 to activate the downstream SPAK/OSR1, resulting in the activation of NCC and NKCC. The activities of NCC and NKCC are also involved in salt reabsorption in the renal tubules, which has a substantial impact on the regulation of the systemic blood pressure. Figure 6: A schematic model of ASK3’s role in the cellular osmotic stress response. When a cell is exposed to hypotonic or hypertonic stress, the cell volume is increased (swelling) or decreased (shrinking), respectively. It is broadly understood that various types of ion channels and transporters are regulated by phosphorylation during the restitution of cell volume. K + -Cl − cotransporter (KCC) is activated by the dephosphorylation in response to cell swelling and releases ions to the outside from the cell to decrease the cell volume. In contrast, NKCC is activated by phosphorylation in response to hypertonic stress and imports ions into the cell to increase the cell volume. Our results suggest that hypotonic stress activates ASK3, leading to the inhibition of the WNK1-SPAK/OSR1 pathway. In contrast, hypertonic stress inhibits ASK3, which relieves WNK1 to activate the downstream SPAK/OSR1, resulting in the activation of NCC and NKCC. The activities of NCC and NKCC are also involved in salt reabsorption in the renal tubules, which has a substantial impact on the regulation of the systemic blood pressure. Full size image The graduated response of ASK3 to osmotic stress could be observed in response to the change of either NaCl or mannitol in the solution ( Fig. 2b and Supplementary Fig. S6 ), suggesting that ASK3 responds to changes not in the NaCl concentration per se , but in the osmolality. The hypotonicity-induced phosphorylation of Thr 808 could not be observed in ASK3 KM ( Fig. 2e ), suggesting that the activation of ASK3 is achieved by autophosphorylation, which may correspond to the autophosphorylation of ASK1 in response to reactive oxygen species [25] . However, it is still unclear what mechanism is involved in the inactivation of ASK3 in hypertonic stress. We are speculating that there should be ASK3 phosphatase(s) activated and/or recruited in response to hypertonic stress. We examined in vitro whether purified ASK3 could directly alter its activity in osmotic solution ( Supplementary Fig. S4 ). Neither the activation in hypotonic solution nor the inactivation in hypertonic solution could be observed for the isolated ASK3. This result suggested that certain cellular components are required to alter the activity of ASK3. The elucidation of the mechanism responsible for the bidirectional regulation of ASK3 is one of the most interesting issues awaiting future studies. We also found that ASK3 functions as a negative regulator of the WNK1-SPAK/OSR1 pathway in the osmotic stress response ( Fig. 3 ). ASK3 knockdown by siRNA resulted in the acceleration of the activity of WNK1 in both HEK293A and HeLa cells ( Fig. 3c ). Additionally, our results suggested that ASK3 suppresses the WNK1-OSR1 pathway through its kinase activity ( Fig. 3e ). The fact that ASK3 depletion affected OSR1 activity in hypotonic stress more than in hypertonic stress further supported the importance of kinase activity in the suppression ( Fig. 3f ). It is conceivable that ASK3-dependent inhibitory regulation counteracts and overrides the activation mechanism of WNK1 in hypotonic stress, whereas WNK1 may be freely activated in hypertonic stress, as ASK3 is inactivated in the hypertonic condition ( Fig. 6 ). The balance between ASK3-independent activation and ASK3-dependent inhibition might determine whether the WNK1-SPAK/OSR1 pathway is activated or inhibited in hypotonic stress. Such hypotonicity-specific inhibition by ASK3 may provide an opportunity for the WNK1-SPAK/OSR1 pathway to be oppositely regulated in hypo- and hypertonic conditions ( Fig. 6 ). Although we have demonstrated the endogenous interaction between ASK3 and WNK1 ( Fig. 3a ) and the importance of the kinase activity of ASK3 ( Fig. 3e ), it is still unknown so far whether ASK3 suppresses WNK1 through the direct phosphorylation of WNK1 or through the phosphorylation of other unidentified protein(s). At least, WNK1 appears to be the pivotal player among the WNK isoforms in the OSR1 hyperactivation induced by ASK3 depletion, because the combinatorial knockdown of WNK1, rather than those of other WNK isoforms, together with ASK3 resulted in the complete abolishment of the effect of ASK3 knockdown ( Fig. 3g and Supplementary Fig. S12 ). Thus, we consider that ASK3 depletion resulted in the OSR1 hyperactivation through the WNK1 misregulation. Therefore, our results propose ASK3 as a novel regulator of the WNK1-SPAK/OSR1 pathway in the osmotic stress response ( Fig. 6 ). Consistent with the cell-based study, we found that the genetic depletion of ASK3 leads to the hyperactivation of SPAK/OSR1 in the kidney ( Fig. 4 ). It is suggested that PHA II patients harbouring genetic mutations of WNK1 or WNK4 and the mouse model of PHA II are affected with hypertension at least in part through the hyperactivation of NCC in the kidney [18] , [30] , [33] , [37] . In the case of WNK1 gene mutation, it is suggested that the mutation causes the overexpression of the WNK1 protein and the misregulation of the splicing of the WNK1 transcript, presumably leading to the hyperactivation of NCC via the abnormally enhanced WNK1-SPAK/OSR1 signaling [18] , [19] , [20] . We considered that the hypertensive phenotype of ASK3 KO mice might be interpretable in a similar context, as hyperphosphorylation of NCC was observed in the kidneys of ASK3 KO mice ( Fig. 4f ). The susceptibility to acute NaCl loading in the maintenance of blood pressure also endorsed the defects in salt homoeostasis in the ASK3 KO mice ( Fig. 5b ). Although it is well established that the patients and mouse model of PHA II are affected not only with hypertension but also with hyperkalemia due to impaired renal K + secretion [18] , [30] , [33] , [37] , ASK3 KO mice exhibit no alteration in the plasma K + concentration and a slight decrease in urinary K + secretion ( P =0.14) ( Supplementary Table S1 ). We suspected that the impact of ASK3 depletion on the renal salt regulation would be milder than that of WNK1 mutation itself, because ASK3 suppresses WNK1 primarily in situations where ASK3 is active, such as in a hypotonic circumstance. The late onset of the mild hypertension in ASK3 KO mice ( Fig. 5a ) may be attributable to the same reason. Alternatively, it is also possible that there might be some ‘back-up’ systems that would maintain plasma K + level under the disruption of ASK3, or ASK3 might exert positive effects on the K + reabsorption independent of its negative effect on the WNK1-SPAK/OSR1 pathway, as ASK3 is also expressed in other renal tubules than the DCT, such as the collecting duct ( Fig. 1e and Supplementary Fig. S2 ). The results presented in our study demonstrate that ASK3 is a unique osmotic stress-responsive kinase that suppresses the WNK1-SPAK/OSR1 pathway in cells and is involved in the control of blood pressure, at least in part through the regulation of SPAK/OSR1 activity in the kidney. Our results also endorse the notion that the hyperactivation of the WNK1-SPAK/OSR1 pathway leads to hypertension from the viewpoint of a novel upstream regulator. Recently, it is suggested by using WNK1 +/− mice that the WNK1-SPAK/OSR1 pathway is involved in the vasoconstriction in the regulation of the systemic blood pressure [31] , [38] . Therefore, it is an interesting issue to investigate whether ASK3 regulates the WNK1-SPAK/OSR1 pathway also in the blood vessels. Further studies on ASK3, including the relationship with other WNK kinases ( Supplementary Fig. S12a ), will provide a novel understanding of the physiological and pathophysiological signal transduction pathways related to body fluid homoeostasis in humans. Antibodies Monoclonal antibodies to human ASK3, mouse ASK3 and human SPAK were established as described previously [23] . GST-tagged C-terminal fragments of human ASK3 (corresponding to amino acids 909–1,313), mouse ASK3 (amino acids 1,085–1,331) and human SPAK (amino acids 340–547) were produced and purified from Escherichia coli strain BL21 as antigens. All of them were used in a 1,000-fold dilution for the immunoblot. The antigen of the monoclonal antibody to phospho-specific ASK (PA41) was constructed by conjugating the synthesized phospho-peptide (amino acids in human ASK3 805–815: CTE[pT]FTGTLQY) with keyhole-limpet hyemcyanin [23] . WYK/Izm rats were immunized via the hind footpads with the recombinant proteins using Freund’s complete adjuvant. The enlarged medial iliac lymph nodes from the rats were used for cell fusion with mouse myeloma cells, SP2, and the hybridoma cells were cultured in GIT medium (Wako Pure Chemicals) supplemented with 100 μM hypoxanthine, 0.4 μM aminopterin, 16 μM thymidine, 10% FBS and 2% BM Condimed H1 (Roche Applied Science). The antibody-secreting hybridoma cells were selected by limiting dilution, screening with enzyme-linked immunosorbent assay and immunoblotting ( Supplementary Fig. S1 ). PA41 was used only in the immunocytochemistry shown in Fig. 2e in a 100-fold dilution. Rabbit polyclonal antibodies to mouse ASK3 (amino acids 201–218: CESDAQRRASEYMQPNWD), P-WNK1 (amino acids 376–388: RASFAK[pS]VIGTPE) and P-SPAK/OSR1 (amino acids 226–239: TRNKVRK[pT]FVGTPC) were constructed as described previously [25] and used in 1,000- (ASK3 and P-WNK1) and 300-fold (P-SPAK/OSR1) dilutions for the immunoblot. P-SPAK/OSR1 antibody was also used in a 500-fold dilution for the immunohistochemistry. The indicated synthetic peptides were conjugated with KLH and used as immunogens. The antisera obtained from immunized rabbits were applied to affinity column for positive selection. The polyclonal antibody to phospho-ASK1 (pT845) was described previously [25] , which was used in all immunoblot experiments as P-ASK antibody in a 2,000-fold dilution. The monoclonal antibody to ASK2 was described previously [23] and used in a 1,000-fold dilution for the immuoblot. The antibody to P-NCC was described and characterized in the previous report [33] , which was used in a 5,000-fold dilution for immunoblot and a 500-fold dilution for immunohistochemistry. The antibody to Flag-tag (M2) and actin (AC-40) were purchased from Sigma and used 500- and 10,000-fold dilutions for the immunoblot, respectively. The antibody to HA-tag (3F10) was purchased from Roche Applied Science and used in a 500-fold dilution for the immunoblot. Phospho-specific antibodies to JNK (P-JNK: Thr 183 /Tyr 185 ), p38 MAPK (P-p38: Thr 180 /Tyr 182 ) and ERK (P-ERK: Thr 202 /Tyr 204 ) were purcased from Cell Signaling and used in 1,000- or 2,000-fold dilutions for the immunoblot. The antibody to ERK was also purchased from Cell Signaling and used in a 1,000-fold dilution for the immunoblot. The antibodies to JNK (JNK-FL) and p38 (C-20-G) were purchased from Santa Cruz Biotechnology and used in 5,000- and 2,000-fold dilutions for the immunoblot, respectively. The antibody to WNK1 was purchased from Bethyl and used in a 5,000-fold dilution for the immunoblot. The antibodies to OSR1 (M06 and M01) were purchased from Abnova and used in a 10,000-fold dilution for the immunoblot. The antibody to tatol-NCC was purchased from Millipore and used in a 500-fold dilution for the immunohistochemistry. Cell culture and osmotic stress treatments HEK293A cells, HeLa cells and MEFs were cultured as described previously [23] . Cells were exposed to osmotic stress by changing the extracellular solutions having three kinds of osmolality (hypotonic, isotonic and hypertonic buffer). Isotonic buffer (300 mOsm per kg H 2 O) contained 130 mM NaCl, 2 mM KCl, 1 mM KH 2 PO 4 , 2 mM CaCl 2 , 2 mM MgCl 2 , 10 mM HEPES, 10 mM glucose and 20 mM mannitol. Hypertonic buffer (500 mOsm per kg H 2 O) contained additional 200 mM mannitol compared with isotonic buffer. In hypotonic buffer (200 mOsm per kg H 2 O), mannitol was excluded and NaCl was reduced to 90 mM from isotonic buffer. The absolute osmolality was verified by a cryoscopic osmometer (OSMOMAT 030; Gonotec). We also used distilled water-diluted culture medium (200 mOsm per kg H 2 O) for hypotonic stimulus. Immunoblotting analysis Cell extracts and immunoprecipitates were resolved on SDS–PAGE and electroblotted onto polyvinylidene difluoride membranes. After blocking with 5% skim milk in TBS-T (50 mM Tris–HCl, 150 mM NaCl and 0.05% Tween 20, pH 8.0), the membranes were probed with appropriate antibodies. The antibody-antigen complexes were detected using the ECL system (GE Healthcare) as described previously [23] . In some experiments, the amount of signals was measured by an image densitometer (ImageJ 1.37v). Immunostaining of the cell and image analyser HEK293A cells were transfected with Flag-tagged ASK3 WT or KM and exposed to osmotic buffer for 20 min. After stimulation, cells were fixed in 4% formaldehyde in PBS, permeabilized in 1% Triton X-100. Blocking was performed with 5% skim milk in TBS-T for 1 h, and then incubated with anti-Flag (M2) and anti-phospho ASK (PA41) antibodies overnight. Then, cells were incubated with secondary antibody (Alexa Fluor 488 anti-rat IgG and Alexa Fluor 555 anti-mouse IgG; Molecular Probes) overnight. Cells were counterstained with Hoechst 33258 (Dojindo) for 3 min before mounting with GEL/MOUNT (Biomeda). Images were collected by a confocal microscope (LSM 510 META; Carl Zeiss). In imaging analysis by ArrayScan VTI (Thermo Scientific Cellomics), sample preparation was identical as described above. Cells were identified by the Hoechst signal in nuclei and ASK3-transfected cells were selected by the Flag signals. The region of interest (ROI) was defined by Flag signal and the fluorescence intensity ratio of P-ASK and Flag (P-ASK/Flag) in the ROI was calculated in each cell to define an ASK3 activity (38–120 cells in each preparation) using Cellomics Collocalization V3 software. Coimmunoprecipitation analysis Coimmunoprecipitation analysis was preformed as described previously [23] . For endogenous proteins, HEK293F cells were lysed with the IP lysis buffer (50 mM Tris–HCl, 150 mM NaCl, 10 mM EGTA, 1% Triton X-100, 1 mM phenylmethylsulfonyl fluoride and 1 μM Leupeptin). The cell extracts were clarified by centrifugation and the supernatants were immunoprecipitated with anti-ASK3 antibody or control rat IgG using Protein G sepharose beads (GE Healthcare). For exogenous tagged protein, HEK293A cells were lysed with the IP lysis buffer. The cell extracts were clarified by centrifugation and the supernatants were immunoprecipitated with Flag antibody gel (M2 gel; Sigma). The beads were washed with the IP lysis buffer before supplied to SDS–PAGE. Immunohistochemistry C57BL/6J strain mice (male, 12-week old) were dissected and the kidney was fixed and embedded in paraffin. Tissue sections were de-paraffined and heat activated in citrate buffer (pH 6.0) for 15 min at 95 °C. After the blocking with ChemMate Anitibody Diluent (Dako), samples were incubated with the monoclonal antibody to mouse ASK3 overnight at 4 °C, and then reacted with Simple Stain MAX-PO (NICHIREI), an amino-acid polymer reagent combined with secondary antibody and peroxidase. Antigen–antibody reaction was visualized with diaminobenzidine tetrahydrochloride and hydrogen peroxide. The samples were counterstained with Mayer’s hematoxylin. The experimental protocol was approved by the Animal Research Committee of the Graduate School of Pharmaceutical Sciences, The University of Tokyo (Tokyo Japan). Cryosection, immunofluorescence and image analysis For the immunofluorescence, the kidneys of age-matched WT and ASK3 KO mice (male, 19–26 weeks old; WT: n =3, KO: n =3) were fixed by perfusion (through the left ventricle) with paraformaldehyde (4%) in PBS as previously described [33] . The tissue samples were soaked for several hours in 20% sucrose in PBS, embedded in Cryo Mount I (Muto Pure Chemicals Co., Ltd.) and frozen in liquid nitrogen. P-SPAK/OSR1 antibody ( Supplementary Fig. S1d ), T-NCC antibody (Millipore) and P-NCC antibody [33] were used as the primary antibodies. When appropriate, λ-phosphatase was administered for 1 h before the primary antibodies. DyLight 546-conjugated anti-rabbit IgG (Jackson ImmunoResearch) was used as the secondary antibody for the immunofluorescence. The immunofluorescence images were obtained with an LSM 510 META (Carl Zeiss) and then analysed using ArrayScan VTI (Thermo Scientific Cellomics) as follows, using Cellomics Collocalization V3 software ( Supplementary Fig. S16 ). The total area of an individual specimen of an image was measured based on the intrinsic fluorescence of the preparation. We carefully obtained images containing the periphery of the kidney to confirm that the objects were in the cortical region. The regions exhibiting stronger fluorescence intensity than a threshold were defined as positive renal tubules, and the summation of these areas was divided by the total area in each specimen to calculate the ratio of positive/total area (%) ( Fig. 4c–e ). We completely analysed 38 images for P-SPAK/OSR1, 18 images for T-NCC and 27 images for P-NCC in each genotype, using three pairs of WT and ASK3 KO mice. Blood pressure measurements In the tail-cuff method, the blood pressure measurements were performed from 20:00 to 00:00, around the start of the dark period of the animal room. The normal blood pressure of unanesthetized mice (ASK3 KO mice or WT littermates; male, 14–30 weeks old) was measured by indirect tail-cuff measurements in every 4 weeks using a BP-98A (Softron). The mice were placed in a cloth holder warmed to 38 °C, and 3–5 consistent measurements (±5 mm Hg between each measurement) were obtained and averaged for each mouse. In the NaCl-loading experiments, the NaCl concentration in the diet was increased from 0.4 to 4% at 0 day under free-feeding conditions (male, 13-weeks-old). The blood pressure was measured at days of −2, 0, 2, 7, 14 and 21 after changing the diet. For the radiotelemetric blood pressure measurements, blood pressure transducers (Data Sciences International) were inserted into the left common carotid artery of age-matched WT and ASK3 KO mice (male, 19–23 weeks old; WT: n =3, KO: n =3). After 1 week of recovery, the values of the systolic and diastolic blood pressure were recorded every minute by telemetry. The mice showed alternating periods of low blood pressure (8:00 to 20:00; the light period) and high blood pressure (20:00 to 8:00; the dark period). For each recording, the blood pressure values were represented by the average for 2 h. At 15 days after the surgery, the mice were fed a high-salt diet (4% NaCl) as a NaCl loading, and the blood pressure values were recorded for 16 more days under free-feeding conditions. Statistical analysis Data are presented as means±s.e.m. Paired means were compared using t -tests. Other methods are presented in the Supplementary information . How to cite this article: Naguro, I. et al . ASK3 responds to osmotic stress and regulates blood pressure by suppressing WNK1-SPAK/OSR1 signaling in the kidney. Nat. Commun. 3:1285 doi: 10.1038/ncomms2283 (2012).